miR828 and miR858 regulate homoeologousMYB2gene functions inArabidopsistrichome and cotton fibre development Although polyploidy is common in plants and some animals, mechanisms for functional divergence between homoeologous genes are poorly understood. MYB2 gene promotes cotton fibre development and is functionally homologous to Arabidopsis GLABROUS1 ( GL1 ) in trichome formation. The most widely cultivated cotton is an allotetraploid ( Gossypium hirsutum , AADD) that contains GhMYB2A and GhMYB2D homoeologs. Here we show that GhMYB2D mRNA accumulates more than GhMYB2A during fibre initiation and is targeted by miR828 and miR858, generating trans -acting siRNAs (ta-siRNAs) in the TAS4 family. Overexpressing GhMYB2A but not GhMYB2D complements the gl1 phenotype. Mutating the miR828-binding site or replacing its downstream sequence in GhMYB2D abolishes ta-siRNA production and restores trichome development in gl1 mutants. Moreover, disrupting Dicer-like protein 4 or RDR6 , the biogenesis genes for ta-siRNAs, in the gl1 GhMYB2D overexpressors restores trichome development. These data support a unique role for microRNAs in functional divergence between target homoeologous genes that are important for evolution and selection of morphological traits. Cotton fibre is not only the largest renewable source of textile materials but also a good model for testing gene functions associated with natural and human selection. The most widely cultivated cotton ( Gossypium hirsutum L., AADD) is an allotetraploid that arose in the New World between the closest relatives of the A-genome species Gossypium herbaceum L. (A1) and Gossypium arboreum L. (A2) and the D-genome species Gossypium raimondii (D5) Ulbrich 1–2 million years ago [1] . Notably, the A-genome species produce spinnable fibre and are cultivated on a limited scale, whereas fibre produced in D-genome species is rudimentary and not useful [2] . The fibre in allotetraploids is much longer and stronger, suggesting non-additive expression (activation or silencing) of homoeologous fibre-related genes. Indeed, some homoeologous genes in allotetraploid cotton exhibit tissue-specific expression patterns [3] , probably through genetic and epigenetic mechanisms [4] , [5] , [6] . Cotton fibre is also a popular model for studying cell differentiation and development. Each cotton fibre is a single-celled seed trichome or hair, and over 20,000 fibres may develop semi-synchronously on each seed. Seed hair development in cotton shares many similarities with leaf trichome development in Arabidopsis [7] . In Arabidopsis thaliana , GLABROUS1 (GL1) is a R2R3 MYB-domain transcription factor and promotes leaf trichome development, which is negatively regulated by TRIPTYCHON (TRY) [8] , [9] . Cotton MYB2 stimulates fibre cell fate determination and is a functional homologue of GL1. Overexpressing G. arboreum MYB2 in A. thaliana complements the glabrous (or trichomeless) mutant gl1 phenotype and induces occasional hair formation in seeds [10] . G. hirsutum RDL1 ( GhRDL1 ) is another fibre-related gene and primarily expressed in seed epidermis and fibre cell initials [11] . Overexpressing both GhMYB2 and GhRDL1 in the A. thaliana try mutant produces seed hair in ~10% of seeds as well as dense trichomes inside and outside siliques. Other fibre-related genes such as GhMYB25 also regulate fibre cell and trichome development in cotton [12] . These data collectively suggest that Arabidopsis and cotton use similar MYB transcription factors for the initiation and development of leaf trichomes and seed hairs. Interestingly, in cotton ovules and fibre many MYB transcripts are targets of microRNAs (miRNAs) including miR828 (ref. 13) [13] , suggesting a role for miR828 in fibre cell development. Small RNAs including miRNAs and trans -acting siRNAs (ta-siRNAs) regulate gene expression and development in plants and animals [14] , [15] . In A. thaliana , biogenesis of ta-siRNAs is often triggered by miRNA cleavage in a TAS locus [16] . The RNA-induced silencing complex associated with ARGONAUTE proteins, AGO1 and AGO7, is recruited to the targeting site to cleave the transcripts [17] . The cleaved mRNA fragment serves as a template for RNA-dependent RNA polymerase6 (RDR6) to generate double-stranded RNAs [18] , [19] , which can be recognized by Dicer-like protein 4 (DCL4) and processed into 21-nt siRNAs in phase or ta-siRNAs [20] . There are eight TAS genes in four families in A. thaliana . Four transcripts in TAS1 and TAS2 families are targeted by miR173 to generate ta-siRNAs that regulate mRNAs including those encoding pentatricopeptide repeat proteins [16] , [18] , [19] . MiR390 triggers cleavage of three TAS3 transcripts following a ‘two-hit’ model [21] . Although miR828 is predicted to target transcripts of several MYB genes [22] , the role for miR828 in MYB gene expression and biogenesis of ta-siRNAs in the TAS4 family is poorly understood. Recent studies indicate that miR828 is induced by sugar and attenuated in abscisic acid in Arabidopsis [23] and wound inducible in sweet potato leaves [24] . Sequencing analysis of degradome found that miR828 targets in maize, rice, grape and apple coincide with the ‘two-hit’ model in the 12-nucleotide interval with miR828 and miR858 (ref. 25) [25] . In this study, we employed the A. thaliana leaf trichome model to test functional roles for miR828 in regulating cotton homoeologous GhMYB2A (originating from A-genome species) and GhMYB2D (originating from D-genome species) genes and their roles in leaf trichome development. Results from a series of genomic, genetic, transgenic and mutant experiments suggest that functional divergence between GhMYB2A and GhMYB2D homoeologous genes is mediated by miR828-directed ta-siRNA production, which regulates leaf trichome development in Arabidopsis and potentially fibre development in cotton. MYB2 genes and their expression in cotton fibres To investigate evolutionary and functional consequences of two MYB2 homoeologous loci in allotetraploid cotton, we cloned and sequenced MYB2 genomic loci from G. hirsutum (AADD) cv. TM-1 and the naked seed mutant N1N1 (AADD), and close relatives of the progenitor species, G. arboreum (A2), G. raimondii (D5) and G. thurberi (D1) ( Fig. 1a and Supplementary Fig. 1 ). These MYB genes contain one intron and are classified into two groups, A- and D-genome like, which were designated MYB2A and MYB2D , respectively ( Fig. 1b ). Between MYB2A and MYB2D sequences, eight single-nucleotide polymorphisms (SNPs) were found in coding regions, one insertion/deletion and multiple nucleotide polymorphisms in the intron ( Supplementary Fig. 1 ). MYB2A coding sequences from all species are identical. Four MYB2D homologues are relatively polymorphic, including five SNPs, leading to non-synonymous mutations in exon 2 (with asterisks, Fig. 1b ). 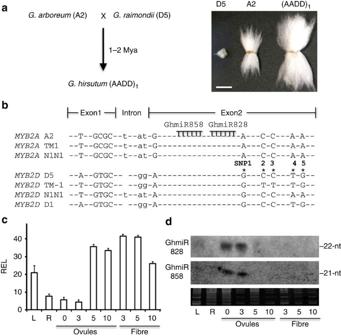Figure 1: Sequence and expression analyses of homoeologousMYB2genes in tetraploid cotton. (a) Cultivated allotetraploid cotton (G. hirsutum, AADD) is formed by polyploidization ~1–2 million years ago between ancestors of A-genome species (G. aboreum, A2) and D-genome species (G. raimondii,D5) (left). The tetraploid cotton has much longer fibres than the progenitors (right). Scale bar, 1 cm. (b) Diagram of alignment using cottonMYB2genomic sequences fromG. arboreum(A2),G. raimondii(D5) andG. hirsutum(AADD, TM-1) and isogenic naked seed mutantN1N1, G. thurberi(D1). SNPs are shown in exons (upper case letters) and introns (lower case letters), and SNPs with non-synonymous mutations inMYB2Dare indicated with asterisks and labelled SNP1, 2, 3, 4 and 5, respectively. miR828 and miR858 binding sites in exon 2 are shown. Lengths of exons and introns are not in the exact scale. Dashes represent identical sequences. (c) qRT–PCR analysis (mean±s.e.m. from three biological replicates) ofGhMYB2expression in TM-1 in tissues of TM-1 leaf (L), root (R) ovules and fibre at 0, 3, 5 and 10 DPA. (d) Small RNA blot analysis of GhmiR828 and GhmiR858 expression. We estimated values of synonymous (Ks) and non-synonymous (Ka) mutations of MYB2 genes ( Supplementary Table 1 ). Synonymous (silent) mutations are largely invisible to natural selection, whereas non-synonymous (amino-acid replacing) mutations may be under strong selective pressure. Ka/Ks ratio can be used as an indicator of selective pressure acting on protein-coding genes, including duplicate genes [26] . Ka/Ks ratios were 0.14 between MYB2A and MYB2D of D1 or N1N1 , 0.18 between MYB2A and MYB2D of D5 and 0.28 among MYB2D homologues ( Supplementary Table 1 ). Higher synonymous mutation rates in MYB2D than in MYB2A suggest stronger selection for MYB2A than for MYB2D . Figure 1: Sequence and expression analyses of homoeologous MYB2 genes in tetraploid cotton. ( a ) Cultivated allotetraploid cotton ( G. hirsutum , AADD) is formed by polyploidization ~1–2 million years ago between ancestors of A-genome species ( G. aboreum , A2) and D-genome species ( G. raimondii, D5) (left). The tetraploid cotton has much longer fibres than the progenitors (right). Scale bar, 1 cm. ( b ) Diagram of alignment using cotton MYB2 genomic sequences from G. arboreum (A2), G. raimondii (D5) and G. hirsutum (AADD, TM-1) and isogenic naked seed mutant N1N1, G. thurberi (D1). SNPs are shown in exons (upper case letters) and introns (lower case letters), and SNPs with non-synonymous mutations in MYB2D are indicated with asterisks and labelled SNP1, 2, 3, 4 and 5, respectively. miR828 and miR858 binding sites in exon 2 are shown. Lengths of exons and introns are not in the exact scale. Dashes represent identical sequences. ( c ) qRT–PCR analysis (mean±s.e.m. from three biological replicates) of GhMYB2 expression in TM-1 in tissues of TM-1 leaf (L), root (R) ovules and fibre at 0, 3, 5 and 10 DPA. ( d ) Small RNA blot analysis of GhmiR828 and GhmiR858 expression. Full size image GhMYB2 was primarily expressed in ovules and fibre in TM-1 ( Fig. 1c ) and in the N1N1 mutant ( Fig. 2a, b ). Previous sequence analysis indicated that MYB2 mRNA was potentially targeted by two miRNAs, GhmiR828 and GhmiR858 in cotton [13] ( Fig. 1b ). In ovules, GhMYB2 was poorly expressed at 0 and 3 days post anthesis (DPA) ( Fig. 1c ), when miR828 and miR858 were most abundant ( Figs 1d and 2c ). In fibre at 3 and 10 DPA, GhmiR828 and GhmiR858 were undetectable in ( Fig. 1d ), which were anti-correlated with high expression levels of GhMYB2 at these stages ( Fig. 1c ). The tissue-specific expression of GhMYB2 in fibre and ovules (but not in leaves or roots) is known under the control of the cis -regulatory elements, including the L1 box in the promoter region [10] , [27] . In leaves, GhMYB2 was expressed ( Figs 1c and 2b , and miR828 was undetectable ( Figs 1d and 2c ). These data suggest that the temporal regulation of GhMYB2 expression during ovule and fibre development is probably mediated by trans -acting factors such as miR828 and miR858 in allotetraploid cotton. 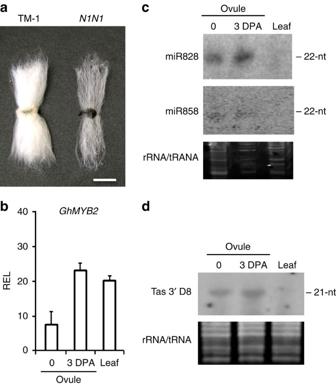Figure 2: miR828, miR858 andMYB2expression in the naked mutant (N1N1) of allotetraploid cotton. (a) Photos of mature seeds with fibres in allotetraploid cotton TM-1 and the isogenicN1N1mutant. Scale bar, 1 cm. (b) REL (mean±s.e.m. from three replicates) ofGhMYB2expression in ovules at 0 and 3 DPA and in leaves of theN1N1mutant. (c) Small RNA blot analysis of miR828 and miR858 in theN1N1mutant in ovules at 0 and 3 DPA and in leaves. (d) Small RNA blot analysis ofGhMYB2-derived ta-siRNAs in theN1N1mutant. rRNA/tRNA was used as a loading control. Figure 2: miR828, miR858 and MYB2 expression in the naked mutant ( N1N1 ) of allotetraploid cotton. ( a ) Photos of mature seeds with fibres in allotetraploid cotton TM-1 and the isogenic N1N1 mutant. Scale bar, 1 cm. ( b ) REL (mean±s.e.m. from three replicates) of GhMYB2 expression in ovules at 0 and 3 DPA and in leaves of the N1N1 mutant. ( c ) Small RNA blot analysis of miR828 and miR858 in the N1N1 mutant in ovules at 0 and 3 DPA and in leaves. ( d ) Small RNA blot analysis of GhMYB2 -derived ta-siRNAs in the N1N1 mutant. rRNA/tRNA was used as a loading control. Full size image GhMYB2D transcripts are preferentially degraded by GhmiR828 MiR828 and miR858 sequences are highly conserved among Arabidopsis , rice, maize and apple [25] . The 22-nt miR828 generates ta-siRNAs belonging to the TAS4 family [22] . Within the mature sequence, GhmiR828 has one nucleotide transition compared with VvmiR828a ( Vitis vinifera , grape) and SsmiR828 ( Salvia sclarea , clary) and two nucleotide transitions relative to AtmiR828 ( A. thaliana ), AlmiR828 ( A. lyrata ) and VvmiR828b ( Fig. 3a ). MiR858 is 21-nt long and differs in two nucleotides and shifts one nucleotide relative to AtmiR858 and AlmiR858 ( Fig. 3b ). Target sites of miR828 and miR858 were predicted in GhMYB2 using the published protocol [16] . The target sites of GhMYB2 homoeologous mRNAs are conserved and separated by 12 nucleotides in the second exon ( Fig. 3c,d ). These binding sites are in the coding region that encodes the helix 3 of the R3 domain of the MYB2 protein ( Supplementary Fig. 1 ). 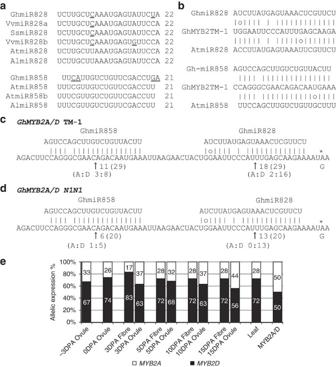Figure 3:GhMYB2transcripts are targeted by miR828 and miR858. (a) Alignment of miR828 and miR858 mature sequences among different plant species, including cotton (Gh,G. hirsutum), grape (Vv,Vitis vinifera), clary (Ss,Salvia sclarea),A. thaliana(At) andA. lyrata(Al). The length of miR828 (22-nt) and miR858 (21-nt) is indicated. Non-conserved sequences are underlined. (b) Comparison ofMYB2transcripts targeted by GhmiR828, AtmiR828, GhmiR858 and AtmiR858. Circles indicate the wobble base pair (U:G). (c) Differential cleavage ofGhMYB2AandGhMYB2Dtranscripts by miR828 and miR858 in TM-1. Arrows indicate cleavage sites. Numbers in the upper row indicate cleaved fragments at miR858 and miR828 sites relative to total fragments tested (in parenthesis). Numbers in the lower row indicate cleavedMYB2AandMYB2Dfragments (A:D) in each site. The asterisk indicates A (MYB2A) to G (MYB2D) transition. (d) Differential cleavage ofGhMYB2AandGhMYB2Dtranscripts by miR828 and miR858 inN1N1. Numbers shown are in the same arrangement as in (c). (e) Pyrosequencing analysis of relative expression levels ofGhMYB2AandGhMYB2Dhomoeologous alleles in allotetraploid cotton in ovules at −3, 0, 3, 5, 10 and 15 DPA, in fibres at 3, 5, 10 and 15 DPA, and in leaves. Figure 3: GhMYB2 transcripts are targeted by miR828 and miR858. ( a ) Alignment of miR828 and miR858 mature sequences among different plant species, including cotton (Gh, G. hirsutum ), grape (Vv, Vitis vinifera ), clary (Ss, Salvia sclarea ), A. thaliana (At) and A. lyrata (Al). The length of miR828 (22-nt) and miR858 (21-nt) is indicated. Non-conserved sequences are underlined. ( b ) Comparison of MYB2 transcripts targeted by GhmiR828, AtmiR828, GhmiR858 and AtmiR858. Circles indicate the wobble base pair (U:G). ( c ) Differential cleavage of GhMYB2A and GhMYB2D transcripts by miR828 and miR858 in TM-1. Arrows indicate cleavage sites. Numbers in the upper row indicate cleaved fragments at miR858 and miR828 sites relative to total fragments tested (in parenthesis). Numbers in the lower row indicate cleaved MYB2A and MYB2D fragments (A:D) in each site. The asterisk indicates A ( MYB2A ) to G ( MYB2D ) transition. ( d ) Differential cleavage of GhMYB2A and GhMYB2D transcripts by miR828 and miR858 in N1N1 . Numbers shown are in the same arrangement as in ( c ). ( e ) Pyrosequencing analysis of relative expression levels of GhMYB2A and GhMYB2D homoeologous alleles in allotetraploid cotton in ovules at −3, 0, 3, 5, 10 and 15 DPA, in fibres at 3, 5, 10 and 15 DPA, and in leaves. Full size image We employed pyrosequencing to quantify expression ratios of GhMYB2A and GhMYB2D endogenous loci. Overall expression levels of GhMYB2D were higher than those of GhMYB2A across all tissues tested. Expression ratios of GhMYB2D to GhMYB2A were 67% in immature ovules at −3 DPA to 83% in young fibre at 3 DPA and maintained at a slightly lower level (72%) during fibre cell elongation ( Fig. 3e and Supplementary Fig. 2a ). Similarly, higher expression levels of GhMYB2D were observed by the analysis of real time polymerase chain reaction (RT–PCR) coupled with cleaved amplified polymorphic sequence (CAPS) ( Supplementary Fig. 2b ). Notably, at 3 DPA, GhMYB2D expression levels were reduced from 83% in fibre to 63% in ovules ( Fig. 3e ), which was coincident with high accumulation of miR828 and miR858 in ovules at this stage ( Figs 1d and 2c ). To test whether GhmiR828 and Ghmi858 cleaves GhMYB2 in cotton, we employed the uncapped 5′ rapid amplification of cDNA ends (5′ RACE) to amplify cleaved products that were subsequently cloned and sequenced. GhMYB2 transcripts were cleaved by both miR828 and miR858 in ovule and fibre tissues of TM-1 and N1N1 ( Fig. 3c,d ). Overall, miR828 generated more cleaved products than miR858 in Texas Marker-1 (TM-1) (18 versus 11 out of 29) and in N1N1 (13 versus 6 out of 20). This is consistent with the ‘two-hit trigger’ model, in which the 5′ site is often but not always cleaved [21] . Among 29 cleaved products within miR828 site, 16 matched GhMYB2D transcripts, and only 2 (12.5%) matched GhMYB2A transcripts in TM-1 ( Fig. 3c ). In the N1N1 mutant, all 13 cleaved products were derived from GhMYB2D transcripts ( Fig. 3d ). Also, miR858-cleaved products were derived more from GhMYB2D than from GhMYB2A transcripts in both TM-1 and N1N1 ( Fig. 3c,d ). Although this method involving ligation and cloning is not straightforward for quantitative analysis, the bias of the cleaved products is probably related to the higher level of GhMYB2D expression. Alternatively, there is a potential preference for miR828 to cleave GhMYB2D transcripts. MYB is a large gene family consisting of 125 R2R3 MYB genes in Arabidopsis [28] and over 240 sequences in the cotton database, Cotton Gene Index 11 (CGI11) [29] . To detect other MYB2 genes that might be targeted by miR828 and miR858 in cotton, we searched the CGI11 database using the two mature miRNA sequences. Five genes are predicted to be miR828 targets, including MYB2 , MYB3 , ATK3 , MYB12, MYB109 and DT461331 ( Supplementary Table 2 ). Among these genes, MYB3 and MYB109 are expressed during fibre development [30] , [31] . However, miR828-directed cleavage products of MYB3 and MYB109 were not amplified in the same mRNA pool used for MYB2 cleavage assays. For miR858, 20 targets were found, including MYB2 , MYB6 , MYB9 , MYB10 , MYB12 , MYB36 and MYB38 ( Supplementary Table 3 ). We could not detect miR858-cleaved products using the candidate target genes TC97370 ( MYB6 ) and TC117537 ( MYB10 ). The data suggest that GhMYB2 is probably the primary target of miR828 during fibre cell development. Production of ta-siRNAs in the TAS4 locus in cotton In addition to the cleavage of target transcripts, miR828 triggers processing of target transcripts into ta-siRNAs [22] , [25] . In the search for small RNA sequences that are derived from cotton ovules and fibres (GEO: GSE16332) [13] , we identified regularly phased ta-siRNAs in GhMYB2 transcripts, initiating from the GhmiR828 cleavage site ( Fig. 4a ) that matched siRNA peaks at positions 3′D2(+), 3′D4(+), 3′D8(+), 3′D9(+) and 3′D10(+) ( Fig. 4b and Supplementary Data 1 ). A phasing register plot showed the graphic display of 21-nt siRNA arrays after the initial cleavage by miR828. The frequency (from 0 to 8) is shown in individual 21-nt intervals (from 1 to 19) ( Fig. 4c ). The phased siRNA distribution analysis revealed that a high proportion of these siRNAs was concentrated in one or two predicted phased positions in the transcripts. Several other cotton MYB homologues, including GhMYB3 , GhMYB109 , GhMYB12 and DT461331 , also generated siRNAs ( Supplementary Fig. 3 ) and siRNA clusters in cotton ovules and fibres ( Supplementary Fig. 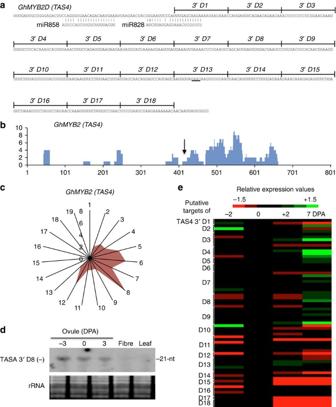Figure 4: GhmiR828-guided cleavage ofGhMYB2transcripts and production of 21-nt phased ta-siRNAs. (a) Diagram of phased ta-siRNA production inGhMYB2Dtranscripts. Sequences of D2′, D4′, D8′, D9′ and D10′ are enriched in cotton small RNA sequencing data. The stop codon is underlined. (b) Small RNA distribution (yaxis, normalized small RNA reads) onGhMYB2transcripts (xaxis: nucleotide position). The arrow indicates the miR828 cleavage site. (c) Phasing registers of ta-siRNAs on cottonGhMYB2exon 2 (456-bp) by miR828. Each spoke of the radial graph indicates the number of 21-nt siRNA matches belonging to one of the 21 possible phasing registers. (d) Small RNA blot analysis of ta-siRNAs generated fromGhMYB2transcripts in cotton (TM-1) ovules at −3, 0, and +3 DPA, fibre at 10 DPA, and leaf. The oligonucleotide probe 3′D8(−) was designed against 3′D8(+). (e) Heat map (green, low and red, high) of relative expression levels for putative targets of ta-siRNAs derived fromGhMYB2transcripts in ovule epidermal cells (−2 to 2 DPA) and fibres (7 DPA) (GSE27506). The expression values were normalized to that at 0 DPA. Putative ta-siRNAs are indicated. 4 and Supplementary Table 4 ) [13] , suggesting that they are potential TAS genes. Figure 4: GhmiR828-guided cleavage of GhMYB2 transcripts and production of 21-nt phased ta-siRNAs. ( a ) Diagram of phased ta-siRNA production in GhMYB2D transcripts. Sequences of D2′, D4′, D8′, D9′ and D10′ are enriched in cotton small RNA sequencing data. The stop codon is underlined. ( b ) Small RNA distribution ( y axis, normalized small RNA reads) on GhMYB2 transcripts ( x axis: nucleotide position). The arrow indicates the miR828 cleavage site. ( c ) Phasing registers of ta-siRNAs on cotton GhMYB2 exon 2 (456-bp) by miR828. Each spoke of the radial graph indicates the number of 21-nt siRNA matches belonging to one of the 21 possible phasing registers. ( d ) Small RNA blot analysis of ta-siRNAs generated from GhMYB2 transcripts in cotton (TM-1) ovules at −3, 0, and +3 DPA, fibre at 10 DPA, and leaf. The oligonucleotide probe 3′D8(−) was designed against 3′D8(+). ( e ) Heat map (green, low and red, high) of relative expression levels for putative targets of ta-siRNAs derived from GhMYB2 transcripts in ovule epidermal cells (−2 to 2 DPA) and fibres (7 DPA) (GSE27506). The expression values were normalized to that at 0 DPA. Putative ta-siRNAs are indicated. Full size image A probe against the MYB2 3′D8(+) sequence was used to detect ta-siRNAs on small RNA blots, and this sequence was selected because of the highest abundance of ta-siRNAs ( Fig. 4c ) and no polymorphism between GhMYB2A and GhMYB2D. We found that ta-siRNAs accumulated at high levels in ovules at 3, 0 and 3 DPA and undetectable in leaves or fibre at 10 DPA ( Figs 2d and 4d ). This ta-siRNA expression pattern was consistent with miR828 abundance levels ( Fig. 1c ). Moreover, microarray expression levels of putative targets (GSE27506) [11] were negatively correlated with target gene expression levels, which were high in fibres at 7 DPA and low in ovules ( Fig. 4e ). These data suggest a potential role for miR828 in generating ta-siRNAs from MYB2 during the development of cotton ovules and fibres. 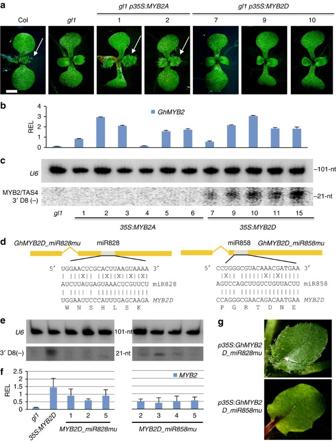Figure 5:GhMYB2Abut notMYB2Dhomoeolog complementsgl1phenotype in transgenicArabidopsis. (a) One-week old seedlings. Trichomes developed (white arrows) in the first two true leaves of the wild type (Col) andgl1transgenic plants expressing35S:MYB2A(#1 and #2) but not in thegl1mutant orgl1transgenic plants expressing35S:MYB2D(#7, #9 and #10). Scale bar, 2 mm for all images. (b) REL(mean±s.e.m. from three replicates) ofGhMYB2expression in Col,gl1and transgenic plants. (c) Small RNA blot analysis of ta-siRNAs derived fromGhMYB2transcripts that accumulated ingl1 35S:MYB2Dtransgenic plants but not ingl1 35S:MYB2Atransgenic plants. Probe was Tas 3′ D8. U6 was used as a control. (d) Diagram ofMYB2Dmutants in the miR828 and miR858 binding sites (indicated by ‘X’) without altering amino-acid sequences. (e) Small RNA blot analysis of ta-siRNAs derived fromGhMYB2transcripts ingl1transgenic plants expressing35S:MYB2D:mR828muand35S:MYB2D:mR858mu, respectively. The same probe as in (c) was used, and U6 was used as a control. (f) REL (mean±s.e.m. from three replicates) ofMYB2expression in transgenic lines shown in (e). (g) Leaf trichome phenotypes in thegl1 35S:MYB2D:mR828mu(white arrow in the upper panel) not ingl1 35S:MYB2D:mR858mu. Search of the cotton database CGI11 and D5 genome [32] identified many putative target genes of MYB2 -derived ta-siRNA, including those encoding sucrose synthase, histone acetyltransferase, glutamate receptor, ethylene-responsive element-binding factor, potassium channel subfamily T, RNA-directed RNA polymerase, F-box containing protein TIR1 and elongation factor ( Supplementary Table 5 and Supplementary Data 1 ) [33] . Some of these genes are known to affect fibre development. For example, SUS3 is involved in fibre cell initiation and elongation [34] , and ethylene is related to fibre cell elongation [35] . GhMYB2A but not GhMYB2D complements the gl1 phenotype To test the function of GhMYB2A and GhMYB2D in the trichome model, we expressed each transgene in the gl1 mutant of A. thaliana . As expected, 35S:GhMYB2A overexpressors in the gl1 mutant restored the trichome development ( Fig. 5a , #1 and #2). However, overexpression of GhMYB2D in the gl1 mutant failed to restore trichomes ( Fig. 5a , #7, #9 and #10). This was surprising because both GhMYB2A and GhMYB2D were highly expressed in these transgenic plants, although their expression levels were variable among multiple independently derived transgenic plants ( Fig. 5b ). The functional divergence between cotton MYB2 homoeologs could be related to trans regulation such as miRNAs and/or protein sequences. Given that GhMYB2 is a TAS4 gene, it is likely that GhMYB2D transcripts were degraded to generate ta-siRNAs. To test this, we examined GhMYB2 -derived ta-siRNAs in these transgenic plants using MYB2/TAS4 3′ D8 as a probe. Indeed, ta-siRNAs accumulated in transgenic lines that expressed 35S:GhMYB2D but not in those that expressed 35S:GhMYB2A ( Fig. 5c ). ta-siRNAs were also detected in ovules but not in leaves ( Fig. 2d ). The data suggest a role for ta-siRNAs in mediating GhMYB2A and GhMYB2D mRNAs that are required for leaf trichome and possibly cotton fibre development. Figure 5: GhMYB2A but not MYB2D homoeolog complements gl1 phenotype in transgenic Arabidopsis . ( a ) One-week old seedlings. Trichomes developed (white arrows) in the first two true leaves of the wild type (Col) and gl1 transgenic plants expressing 35S:MYB2A (#1 and #2) but not in the gl1 mutant or gl1 transgenic plants expressing 35S:MYB2D (#7, #9 and #10). Scale bar, 2 mm for all images. ( b ) REL(mean±s.e.m. from three replicates) of GhMYB2 expression in Col, gl1 and transgenic plants. ( c ) Small RNA blot analysis of ta-siRNAs derived from GhMYB2 transcripts that accumulated in gl1 35S:MYB2D transgenic plants but not in gl1 35S:MYB2A transgenic plants. Probe was Tas 3′ D8. U6 was used as a control. ( d ) Diagram of MYB2D mutants in the miR828 and miR858 binding sites (indicated by ‘X’) without altering amino-acid sequences. ( e ) Small RNA blot analysis of ta-siRNAs derived from GhMYB2 transcripts in gl1 transgenic plants expressing 35S:MYB2D:mR828mu and 35S:MYB2D:mR858mu , respectively. The same probe as in ( c ) was used, and U6 was used as a control. ( f ) REL (mean±s.e.m. from three replicates) of MYB2 expression in transgenic lines shown in ( e ). ( g ) Leaf trichome phenotypes in the gl1 35S:MYB2D:mR828mu (white arrow in the upper panel) not in gl1 35S:MYB2D:mR858mu. Full size image MiR828 regulates GhMYB2A and GhMYB2D expression in vivo GhmiR828 targets GhMYB2 in cotton. However, GL1, a MYB2 homologue in Arabidopsis , does not contain any sequence feature that could be targeted by miR828 from either Arabidopsis or cotton. As a result, A. thaliana is a good system for testing cotton GhmiR828 and GhMYB2 functions in vivo . To test whether miR828 directly degrades GhMYB2D transcripts, we mutated the miR828- and miR858-targeting sites of GhMYB2D , without changing their amino-acid sequences ( Fig. 5d ). The resulting GhMYB2D constructs were transformed into the gl1 mutants. In gl1 transgenic plants expressing 35S:GhMYB2D_miR828mu , MYB2D accumulation ( Fig. 5f ), and ta-siRNAs were undetectable ( Fig. 5e ). This is probably related to the mutated target site, which blocked ta-siRNA cleavage. Consequently, trichomes were recovered in the gl1 transgenic plants expressing 35S:GhMYB2D_miR828mu transgenic lines ( Fig. 5g ). These data imply that 35S:GhMYB2D transcripts are targeted by miR828 in the A. thaliana gl1 mutant that triggers ta-siRNA formation and prevents them from functioning in trichome development. In the gl1 transgenic plants expressing 35S:GhMYB2D_miR858mu , ta-siRNA levels were produced at a reduced level ( Fig. 5e ), but trichome was not restored ( Fig. 5g ). The role of miR858 is probably to assist miR828 targeting, which needs further investigation. GhMYB2A restored trichome development in the gl1 mutants ( Fig. 6a ). To test if the function of GhMYB2A in trichome development is controlled by cotton miR828, we co-transformed gl1 35S:GhMYB2A plants with another transgene 35S:GhamiR828 ( Fig. 6a , #2, #3, and #6). Among multiple independently derived transgenic plants, trichomes were nearly absent in some plants (#6) and reduced in other plants (#2 and #3). The most severe reduction of trichomes correlated with the highest level of GhmiR828 in plant #6 ( Fig. 6b ), but MYB2 expression levels were similar among these transgenics ( Fig. 6d ). As controls, overexpressing GhamiR828 alone in gl1 mutants did not alter trichome phenotypes ( Fig. 6a ). 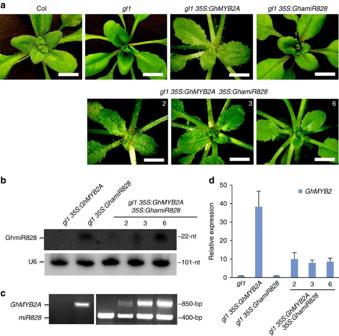Figure 6: Suppression of trichome development by overexpressing GhamiR828 ingl135S:GhMYB2Atransgenic plants. (a) Leaf trichome phenotypes in Col-0 wild type,gl1mutant,35S:GhMYB2Aingl1,35S:GhamiR828ingl1,coexpression of35S:GhMYB2and35S:GhamiR828ingl1(#2, #3 and #6). Scale bar, 5 mm for all images. (b) Small RNA blot analysis of miR828 in the plants as in (a). U6 was used as a control. (c) Genomic DNA PCR amplification of the transgenes35S:GhMYB2Aand35S:GhamiR828inserts in the transgenic plants as in (b). (d) Relative expression levels (mean±s.e.m. in three replicates) ofGhMYB2expression levels in the plants as in (a). Figure 6: Suppression of trichome development by overexpressing GhamiR828 in gl1 3 5S:GhMYB2A transgenic plants. ( a ) Leaf trichome phenotypes in Col-0 wild type, gl1 mutant, 35S:GhMYB2A in gl1 , 35S:GhamiR828 in gl1, coexpression of 35S:GhMYB2 and 35S:GhamiR828 in gl1 (#2, #3 and #6). Scale bar, 5 mm for all images. ( b ) Small RNA blot analysis of miR828 in the plants as in ( a ). U6 was used as a control. ( c ) Genomic DNA PCR amplification of the transgenes 35S:GhMYB2A and 35S:GhamiR828 inserts in the transgenic plants as in ( b ). ( d ) Relative expression levels (mean±s.e.m. in three replicates) of GhMYB2 expression levels in the plants as in ( a ). Full size image Overexpressing MYB2D in ta-siRNA mutants restores trichomes Biogenesis of ta-siRNAs requires RDR6 and DCL4 (refs 18 , 19 , 20 , 36 ). To further test whether disrupting the ta-siRNA biogenesis pathway alters the function of GhMYB2D , we crossed gl1 35S:GhMYB2D transgenic plants that lacked trichomes because of ta-siRNA formation, with the mutant rdr6-11 or dcl4-2 . RDR6 is required for juvenile development, and in the rdr6 mutant, trichomes develop in the abaxial side on the third leaf [19] . To avoid this side effect, we examined adaxial leaf trichomes in 2-week-old seedlings with three pairs of visible juvenile leaves ( Supplementary Fig. 5a ). Genotyping analysis of individual plants in segregating populations identified two 35S:GhMYB2D lines that contained homozygous gl1 and rdr6-11 loci and three 35S:GhMYB2D lines that were homozygous at gl1 and dcl4-2 loci ( Fig. 7a ). Trichome development was restored in two transgenic 35S:GhMYB2D plants that were homozygous at the gl1 and rdr6-11 loci ( Fig. 7a ), probably due to GhMYB2D expression ( Fig. 7b ), as a result of disrupting ta-siRNA biogenesis in the mutant backgrounds ( Fig. 7c ). Similarly, trichome development was restored in three independently derived transgenic 35S:GhMYB2D plants that were homozygous at the gl1 and dcl4-2 loci ( Fig. 7a ), which correlated with activation of GhMYB2D expression ( Fig. 7d ) and low abundance of ta-siRNAs in these plants ( Fig. 7e ). As controls, leaf trichomes developed normally in rdr6-11 35S:GhMYB2D and dcl4-2 35S:GhMYB2D lines because GL1 was present ( Fig. 7a and Supplementary Fig. 5 ). No trichomes were found in rdr6-11 gl1 and dcl4-2 gl1 double mutants, similar to that in the gl1 mutant. In the dcl4-2 gl1 double mutant, purple leaves were found in dcl4-2 mutant as previously described [19] , but no trichomes were observed ( Supplementary Fig. 5 ). 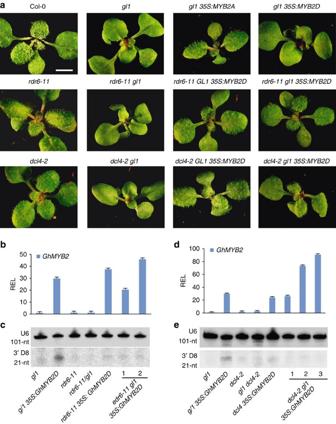Figure 7: Trichome development is restored ingl1 35S:MYB2Dtransgenic plants homozygous forrdr6-11ordcl4-2. (a) Glabrous phenotypes in thegl1mutant andgl1 35S:MYB2Dtransgenic lines; reactivation of trichomes inrdr6-11/gl1 35S:MYB2Dtransgenic plants; reactivation of trichomes ingl1/ dcl4-2 35S:MYB2Dtransgenic plants. Scale bar, 3 mm for all images. (b) REL (mean±s.e.m. from three replicates) ofGhMYB2expression inA. thaliana gl1, andgl1 rdr6-11mutants and transgenic plants expressing 35S:MYB2D. (c) Small RNA blot analysis of ta-siRNA derived fromGhMYB2transcripts inA. thalianamutants and transgenic plants expressing 35S:MYB2D. The same materials were used as in (b). The probe was Tas 3′ D8, and U6 was used as a control. (d) REL (mean±s.e.m. from three replicates) ofGhMYB2expression inA. thaliana gl1,dcl4-2 rdr6-11mutants and transgenic plants expressing 35S:MYB2D. (e) Small RNA blot analysis of ta-siRNA derived fromGhMYB2transcripts inA. thalianamutants and transgenic plants expressing 35S:MYB2D. The same materials were used as in (d). Figure 7: Trichome development is restored in gl1 35S:MYB2D transgenic plants homozygous for rdr6-11 or dcl4-2. ( a ) Glabrous phenotypes in the gl1 mutant and gl1 35S:MYB2D transgenic lines; reactivation of trichomes in rdr6-11/gl1 35S:MYB2D transgenic plants; reactivation of trichomes in gl1/ dcl4-2 35S:MYB2D transgenic plants. Scale bar, 3 mm for all images. ( b ) REL (mean±s.e.m. from three replicates) of GhMYB2 expression in A. thaliana gl1 , and gl1 rdr6-11 mutants and transgenic plants expressing 35S: MYB2D . ( c ) Small RNA blot analysis of ta-siRNA derived from GhMYB2 transcripts in A. thaliana mutants and transgenic plants expressing 35S: MYB2D . The same materials were used as in ( b ). The probe was Tas 3′ D8, and U6 was used as a control. ( d ) REL (mean±s.e.m. from three replicates) of GhMYB2 expression in A. thaliana gl1 , dcl4-2 rdr6-11 mutants and transgenic plants expressing 35S: MYB2D . ( e ) Small RNA blot analysis of ta-siRNA derived from GhMYB2 transcripts in A. thaliana mutants and transgenic plants expressing 35S: MYB2D . The same materials were used as in ( d ). Full size image SNPs affect the function of GhMYB2 homoeologs The specificity of miR828 for targeting GhMYB2D transcripts led us to test if GhMYB2D and GhMYB2A transcripts are degraded differently, leading to functional divergence. GhMYB2A and GhMYB2D have identical mature miR828-binding sites, but there is a SNP, located 4-bp downstream of the miR828-binding site ( Fig. 1b and Supplementary Fig. 1 ). To test the consequence of this sequence difference, we made four chimeric constructs, named Chi1–4 ( Fig. 8a and Supplementary Table 6 ). In Chi1, the amino terminus GhMYB2A was fused into the carboxy terminus GhMYB2D (including SNP1 from GhMYB2D ), whereas in Chi2, the N terminus GhMYB2D was fused into the C terminus GhMYB2A (including SNP1 from GhMYB2A ). In Chi3, SNP1 in GhMYB2A was replaced with that in GhMYB2D , whereas in Chi4, SNP1 in GhMYB2D was replaced with that in GhMYB2A . These constructs were transformed into the gl1 mutant, respectively, and the number of transgenic lines that produced trichomes in 2-week-old rosette leaves was counted. The leaves with trichomes, if present, were harvested for gene expression and small RNA blot analysis. 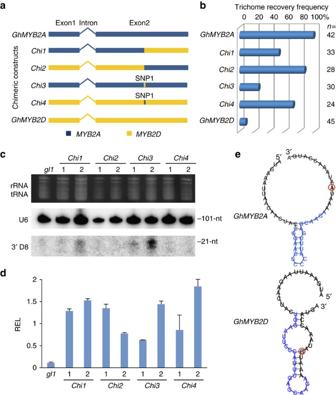Figure 8: Functional tests ofGhMYB2AandGhMYB2Dhomoeologs in trichome development. (a) Diagram of chimerical constructs (Chi1–4) that were used to test functional effects of miR828-targeting sites ofGhMYB2homoeologs on trichome development. (b) Frequency (%) of trichome recovery ingl1transgenic plants expressingGhMYB2A,GhMYB2Dand chimeric constructs. The number of transgenic plants (n) surveyed is shown in the right. (c) Small RNA blot analysis of ta-siRNAs derived fromGhMYB2transcripts ingl1transgenic plants expressing Chi1-4 constructs, respectively. Two independent transgenic plants were analysed for each of Chi1-4. Tas 3′ D8 was used as a probe. U6 RNA blot and rRNA/tRNA gel images were used as RNA loading controls. (d) qRT–PCR analysis ofMYB2expression levels (mean±s.e.m. from three replicates) in the transgenic plants in (c). (e) Predicted secondary structures ofGhMYB2AandGhMYB2DRNA near the miR828-binding region. Red circle indicates SNP1 position, and blue highlights the miR828-targeting site. Figure 8: Functional tests of GhMYB2A and GhMYB2D homoeologs in trichome development. ( a ) Diagram of chimerical constructs (Chi1–4) that were used to test functional effects of miR828-targeting sites of GhMYB2 homoeologs on trichome development. ( b ) Frequency (%) of trichome recovery in gl1 transgenic plants expressing GhMYB2A , GhMYB2D and chimeric constructs. The number of transgenic plants ( n ) surveyed is shown in the right. ( c ) Small RNA blot analysis of ta-siRNAs derived from GhMYB2 transcripts in gl1 transgenic plants expressing Chi1-4 constructs, respectively. Two independent transgenic plants were analysed for each of Chi1-4. Tas 3′ D8 was used as a probe. U6 RNA blot and rRNA/tRNA gel images were used as RNA loading controls. ( d ) qRT–PCR analysis of MYB2 expression levels (mean±s.e.m. from three replicates) in the transgenic plants in ( c ). ( e ) Predicted secondary structures of GhMYB2A and GhMYB2D RNA near the miR828-binding region. Red circle indicates SNP1 position, and blue highlights the miR828-targeting site. Full size image In Chi3 transgenic plants, replacing the miR828-binding site including SNP1 of GhMYB2D with that of GhMYB2A dramatically reduced trichome development (in only 20% of plants) ( Figs 8b and 9 ), and ta-siRNAs were detected in leaves of two transgenic plants tested ( Fig. 8c ). In the gl1 transgenic plants expressing the construct Chi4, ta-siRNAs were undetectable, and trichome development was restored in 65% of the plants. Replacing C terminus of GhMYB2D with that of GhMYB2A in Chi2 transgenic plants restored trichome development in 80% of the plants ( Figs 8b and 9 ). However, in the reciprocal swapping experiment with Chi1 (containing SNP1 of GhMYB2D ), trichome development was still present in only ~42% of the plants, which correlated with production of variable ta-siRNAs in the two lines tested ( Fig. 8c ). In some lines, MYB2 expression levels did not correlate well with ta-siRNA accumulation levels ( Fig. 5c,d ). Although GhMYB2 expression levels were variable among these Chi transgenic lines tested, presence or absence of trichome was anti-correlated with ta-siRNA production. The data suggest that cleavage of GhMYB2 transcripts by miR828 is necessary but not sufficient for trichome development. Other factors such as non-synonymous mutations in the C terminus of GhMYB2A may also play a role for GhMYB2 in trichome development. 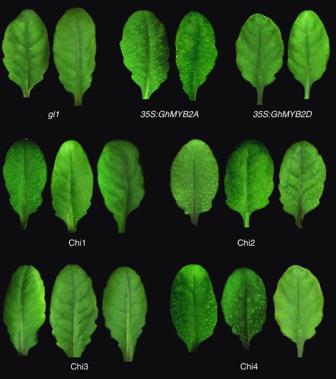Figure 9: Trichome phenotypes in the transgenic plants that expressed chimeric sequences betweenGhMYB2AandGhMYB2D. Images of the fifth rosette leaf were shown in thegl1mutant andgl1transgenic plants expressing35S:GhMYB2A,35S:GhMYB2D, Chi1, Ch2, Ch3 and Ch4, respectively. Diagrams of Chi1-4 constructs are shown inFig. 8. Figure 9: Trichome phenotypes in the transgenic plants that expressed chimeric sequences between GhMYB2A and GhMYB2D . Images of the fifth rosette leaf were shown in the gl1 mutant and gl1 transgenic plants expressing 35S:GhMYB2A , 35S:GhMYB2D , Chi1, Ch2, Ch3 and Ch4, respectively. Diagrams of Chi1-4 constructs are shown in Fig. 8 . Full size image One hypothesis for this functional divergence is that the SNP caused an unpaired base in the targeting site and led to a looser secondary structure and a lower energy cost. This could have increased miRNA site accessibility and promoted its target mRNA degradation [37] , [38] . To test the hypothesis, we predicted mRNA secondary structures of GhMYB2 homoeologs using Vienna RNAfolder (RNAfold WebServer, http://www.rna.tbi.univie.ac.at/cgi-bin/RNAfold.cgi ). Analysing the minimum free energy in the sequences that flank 17 nucleotides upstream and 13 nucleotides downstream of the miR828-binding site, we found that SNP1 resulted in a subtle difference on the free energy of binding (−17.03 kcal mol −1 of MYB2A and −16.09 kcal mol −1 of GhMYB2D ) within this region, which could alter the mRNA secondary structure in miRNA-binding regions of GhMYB2A and GhMYB2D ( Fig. 8e ). Although the prediction may not reflect the RNA-folding in vivo , this structural alteration is predicted to affect accessibility of miR828 to the complementary cleavage site of mRNA targets, which may lead to the observed cleavage difference between GhMYB2A and GhMYB2D transcripts. Polyploidy (whole-genome duplication) is a prominent evolutionary feature in many flowering plants and some animals [39] . Many important crops such as wheat and cotton are polyploids containing two or more sets of chromosomes. These extra sets of genetic materials and/or increased levels of heterozygosity in polyploids are predicted to be advantageous for selection, adaption and domestication [40] , [41] . Polyploidy induces non-additive expression of homoeologous genes [4] , [5] , [6] , through mechanisms of transcriptional regulation via chromatin modifications [42] and DNA methylation [43] , [44] , posttranscriptional regulation involving small RNA regulation [45] , [46] , [47] , mRNA stability in Arabidopsis allotetraploids [48] , alternative splicing in Brassica allotetraploids [49] and posttranslational modifications in allopolyploids of Arabidopsis [50] and Brassica [51] . Functional divergence between MYB2 homoeologs is a good example of the miRNA-mediated mechanisms for evolutionary and functional consequences of duplicate genes in polyploids ( Fig. 10 ). This miRNA-mediated target specificity is an attractive mode for regulating homoeologous transcripts originating from different species. 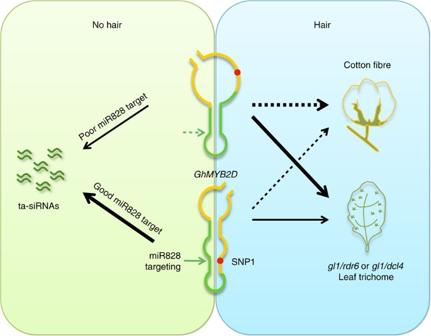Figure 10: A model for miR828-mediatedMYB2homoeologous gene divergence in trichome and fibre development. BothGhMYB2AandGhMYB2Dproteins can promote development of fibre cells in cotton and trichomes inArabidopsis.In cells that do not produce trichomes or fibres, miR828 is highly expressed, andGhMYB2AandGhMYB2Dare degraded into ta-siRNAs. The target site in theGhMYB2AmRNA may be poorly accessible to miR828 (green dashed arrow), whereas the target site located between two bulges inGhMYB2Dis highly accessible to miR828 (green arrow), which leads to degradation ofGhMYB2Dand ta-siRNA production. In cells that produce trichome and fibres,GhMYB2Ais functional and promote trichome or fibre development. When the ta-siRNA pathway is mutated, trichome is restored. In addition,GhMY2Doriginates from progenitors with rudimentary fibres, and mutations accumulate over time. As a result,GhMYB2Dalone may function poorly in promoting trichome and fibre development. Diagrams of a leaf with trichomes and a cotton boll with fibre are shown. Short waved lines: ta-siRNAs; red circles: location of SNP1; black arrows: pathways supported by the data; dashed arrows: predicted function; fat and thin lines: relative levels of targeting or contribution to the trait. Figure 10: A model for miR828-mediated MYB2 homoeologous gene divergence in trichome and fibre development. Both GhMYB2A and GhMYB2D proteins can promote development of fibre cells in cotton and trichomes in Arabidopsis. In cells that do not produce trichomes or fibres, miR828 is highly expressed, and GhMYB2A and GhMYB2D are degraded into ta-siRNAs. The target site in the GhMYB2A mRNA may be poorly accessible to miR828 (green dashed arrow), whereas the target site located between two bulges in GhMYB2D is highly accessible to miR828 (green arrow), which leads to degradation of GhMYB2D and ta-siRNA production. In cells that produce trichome and fibres, GhMYB2A is functional and promote trichome or fibre development. When the ta-siRNA pathway is mutated, trichome is restored. In addition, GhMY2D originates from progenitors with rudimentary fibres, and mutations accumulate over time. As a result, GhMYB2D alone may function poorly in promoting trichome and fibre development. Diagrams of a leaf with trichomes and a cotton boll with fibre are shown. Short waved lines: ta-siRNAs; red circles: location of SNP1; black arrows: pathways supported by the data; dashed arrows: predicted function; fat and thin lines: relative levels of targeting or contribution to the trait. Full size image In this study, we tested the function of homoeologous genes in cotton fibre development using the heterologous trichome cell model. The functional divergence between GhMYB2 homoeologous genes is a good example of cis and trans -regulation [52] . The promoter activity of G. arboreum MYB2 is restricted in leaf trichomes and cotton fibre cells [27] . This cis -acting effect on allelic expression bias is similar in leaves to that in ovules and fibres, although MYB2 expression is very low in vegetative tissues such as leaves and roots [10] . However, trans -regulation involving miR828 and miR858 determines the functional difference between GhMYB2A and GhMYB2D homoeologous genes in Arabidopsis leaf trichomes and possibly cotton fibres. Other factors that are absent in Arabidopsis leaves could also play roles in cotton fibre cell development. Additional data on transgenic cotton could rule out a possibility that GhMYB2D may also contribute to fibre development. Differential cleavage of homoeologous transcripts in Arabidopsis allotetraploids has been previously observed [46] . In one example, cis- and trans -regulation of A. thaliana and A. arenosa miR163 mediates expression of homoeologous target genes responsible for secondary metabolites with a potential role in defence response [50] . Transcription of A. arenosa MIR163 is repressed, and processing efficiency for mature A. arenosa miR163 is also low, leading to accumulation of downstream target transcripts. Compared with A. thaliana miR163, A. arenosa miR163 has a poor efficiency of target cleavage, as occurred for other miRNAs such as miR164, miR168 and miR172 (ref. 46) [46] . The process of miRNA binding to the target site is determined by both the binding site and flanking sequence [37] , [53] . In humans, miR-223 targets 3′ untranslated region of RhoB mRNA, and AU-rich motif at 5′ upstream of miR-223-targeting site affects miR-223 accessibility [54] . In plants including Arabidopsis , rice, maize and grape, sequences near the miRNA-targeting sites affect both accessibility and function of miRNAs to their target transcripts [38] . Our data suggest that the sequence variation near the miR828-targeting site determine the ta-siRNA production and functional difference between GhMYB2A and GhMYB2D . The sequence changes near the miRNA-targeting site alter the mRNA secondary structure in GhMYB2D , increasing miRNA accessibility and subsequently GhMYB2D transcript degradation. These data support the prediction that secondary structures near the miRNA-targeting site are critical for degradation of target mRNA [46] , [47] , which offer another mechanism for differential expression of homoeologous genes in Arabidopsis and other allopolyploid plants. In addition to miRNA target regulation, non-synonymous changes in other regions between GhMYB2A and GhMYB2D homoeologs may also affect protein functions and lead to functional divergence in trichome and fibre development. GhMYB2A is under stronger selection than GhMYB2D because fibre production is selected in G. arboreum -like species where GhMYB2A originates, while the function of GhMYB2D resembles its fibreless progenitors probably due to miR828 targeting and sequence mutations. Our data suggest that TAS4 itself encodes a MYB transcription factor that is important to the cellular process of trichome formation in Arabidopsis and possibly fibre development in cotton. TAS4 is inducible by sugar [55] . In cotton, one might predict a role of TAS4 in suppressing carbohydrate metabolism including sucrose and cellulose, which are required for fibre development; instead, diverting carbon sources to promote other physiological and metabolic activities essential for general plant growth and development. Changes in the secondary structure near the miR828-binding site may result from coevolution between miRNA and target gene sequences. As a result, GhMYB2D is more promiscuously degraded by miR828 cleavage than GhMYB2A . Cotton miR828 also recognizes and cleaves GhMYB2D transcripts but not GhMYB2A transcripts in A. thaliana . In cotton, fibre develops well in A-genome species but poorly in D-genome species such as G. raimondii . This could be related to preferential degradation of GrMYB2 transcripts by miR828 and/or non-synonymous mutations in the GrMYB2 gene. In allotetraploid cotton, there is a paradox that many quantitative trait loci are associated with D-genome [56] , and gene expression is also biased towards D-genome [57] . This paradox could be explained in part by some negative regulators including small RNAs that suppress one of the homoeologous transcripts such as GhMYB2D that is associated with poor fibre traits at the posttranscriptional level. Natural selection and human domestication could have enhanced this potential of using ‘better’ genes for ‘superior’ traits. This mechanism for differential targeting and degradation of homoeologous transcripts could be a result of coevolution between miRNAs and their target genes that control morphological traits like fibre and adaptive traits like defence response. Plant material G. hirsutum L. cv. TM-1, the near-isogenic N1N1 mutant in TM-1, G. arboretum (A2), G. thurberi (D1) were grown in a greenhouse at 30 to 35 °C under natural light supplemented with fluorescent illumination in a daily cycle of light (16 h) and dark (8 h). Cotton flowers on the day of anthesis (0) were tagged, and the bolls were harvested at specified DPA. For cotton ovules prior to anthesis (for example, −3 DPA), the time of flowering was estimated based on flower position and size, and ovules were harvested. Harvested tissues were stored on ice until dissection, and the ovules with fibre were carefully dissected from each boll. Cotton fibres (3–15 DPA) were isolated from ovules by gently grounding in liquid nitrogen, and stored at −80 °C for nucleic acid extraction. Tissues of G. raimondii (D5) were provided by David Stelly at Texas A&M University. A. thaliana Columbia 0 (Col-0), gl1-1 (CS1644) and rdr6-11 (CS24285) mutants were obtained from the Arabidopsis Biological Resource Center. The dcl4-2 was kindly provided by Zhixin Xie at Texas Tech University [20] . Arabidopsis plants were grown in a growth chamber at 22 °C with a daily cycle of light (16 h) and dark (8 h). Genotyping of the gl1-1 mutant (CS1644) was performed based on a single-nucleotide mutation at position 1305 of the GL1 locus (AF263690). The PCR primer pair used for CAPS analysis was AtGL1-DdeI-R1, 5′-ATCTGTTCTTCCCGGTACTCTTTTAGCTATCTAA-3′; and AtGL1-F2, 5′-GTTAGAAACGTTTTCCACAATTG-3′, which were designed according to the website ( http://www.helix.wustl.edu/dcaps/dcaps.html ). The amplified fragments were 234-bp in size and digested into 201-bp and 33-bp fragments by Dde I in the wild type, but not in the mutant. The primers for PCR detection of T-DNA insertion mutants in dcl4-2 were: DCL4-F, 5′-GCTCATGAGAACATAACAACCT-3′, DCL4-R, 5′-TTCGTGCAAGAGGGATTTT-3′ and LBb1 primer, 5′-GCGTGGACCGCTTGCTGCAACT-3′. Genomic identification of rdr6-11 used PCR amplification with the primer pair: RDR6-F, 5′-TACTGTCCCTGGCGATCTCT-3′ and RDR6-R, 5′-CCACCTCACACGTTCCTCTT-3′, followed by digestion with the restriction enzyme Taq I. There are three fragments (15-bp, 79-bp and 93-bp) in the wild type and two fragments (79-bp and 108-bp) in the mutant. Cloning and plant transformation The MYB2 sequence was amplified from cotton genomic DNA using the primer pair of XhoI-GhMYB2-F, 5′-CTCGAGATGGCTCCAAAGAAGGATG-3′ and NotI-GhMYB2-R, 5′-GCGGCCGCTTATACCATTGCTAATGG-3′. The PCR products were ligated into the pGEMT vector and sequenced. The MYB2 fragment was then subcloned into the binary vector pBARN. Two rounds of PCR reaction were conducted using specific primer pair and template plasmid DNA with GhMYB2A or GhMYB2D . Round I was to amplify the chimerical fragments, and round II was to amplify the entire chimerical GhMYB2 fragment using the primer pair of Xho I-GhMYB2-F, 5′-CTCGAGATGGCTCCAAAGAAGGATG-3′ and Not I-GhMYB2-R, 5′-GCGGCCGCTTATACCATTGCTAATGG-3′ and using PCR products of the round I as the template DNA. The primers used for chimerical constructs are list in Supplementary Table 6 . The insert sequence was confirmed by digestion with Xho I and Not I and ligated into the binary vector pBARN under the 35S promoter. The GhmiR828 mature sequence was cloned into the miR159a plasmid using the published method [58] . Specifically, the sequence of the A. thaliana miR159a precursor was cloned by PCR amplification using primers XhoI-miR159-F1 (5′-CTCGAGCACCACAGTTTGCTTATGTCGGATCC-3′) and NotI-miR159-R1 (5′-GCGGCCGCATG TAGAGCTCCCTTCAATCC -3′). The PCR fragment was cloned into pGEMT vector (Promega) by TA cloning. Mutagenesis of pre-miR159a was performed by PCR using amiR828-F1 and amiR828-R1 primers. The amiR828-F1 primer (5′-AAGAT AGATCT TGATCTGACGATGGAAG TCTTGCTCAAATGAGTATTCTA CATGAGTTGAGCAGGGTA-3′) contains a Bgl II site (italic) and the amiR828* sequence (underlined). The amiR828-R1 primer (5′- GCGGCCGC ATG TCTTGCTCAAATGAGTATTCTA GAAGAGTAAAAGCCATTA-3′) contains a Not I site (italic) and the mature amiR828 reverse complementary sequence (underlined). pGEMT-pre-miR159a DNA was used as a template for PCR mutagenesis. The resulting DNA fragment was subsequently digested with Bgl II and Not I and inserted into pGEMT-pre-miR159a to generate pGEMT-pre-amiR828. The mutations introduced can form the fully complementary miRNA:miRNA* pair. Finally, the pGEMT-pre-amiR828 vector DNA was digested with Xho I and Not I, and the resulting fragments were ligated into the binary vector pBARN for plant transformation. The final artificial miRNA insert was cloned into pBARN vector. The constructs were transformed into the Agrobacterium strain GV 3101 that was transformed into A. thaliana Col-0 using the floral dip method [59] . Estimation of Ka and Ks values Exon 2 sequences, where SNPs are present, of three MYB2A alleles from A2, TM-1, N1N1 genotypes, and four MYB2D alleles from D1, D2, N1N1, TM-1 genotypes were aligned by CLUSTAL W using default parameters. The number of synonymous and non-synonymous substitution sites was estimated using MEGA5 with the Nei–Gojobori Method and the Jukes–Cantor Model ( http://www.megasoftware.net/mega.php ). The Ka/Ks ratio was calculated using numbers of synonymous/non-synonymous substitution sites. CAPS analysis MYB2 fragments were amplified by PCR using the primer pair of CAP-MYB2-F:5′-ATGGCTCCAAAGAAGGATGGAG-3′ and CAP-MYB2-R: 5′-TCATTGTCTGGTCGCCCTGGA)-3′ and digested by Hha I. The length of genomic fragments of GhMYB2 was 387-bp, and the products from GhMYB2A were digested to yield 290-bp and 97-bp fragments. The length of cDNA fragments in GhMYB2 was 310-bp. GhMYB2A cDNA fragments were digested to yield two fragments (213-bp and 97-bp). GhMYB2D fragments cannot be digested by Hha I. Pyrosequencing analysis of GhMYB2 homoeologs PCR primers and sequencing primers were designed and checked with Pyro Mark Assay Design software, CAPS-MYB2-F_Biotin_tag, 5′-GCTCCAAAGAAGGATGGAGTG-3′, CAPS-MYB2-R1, 5′-TGTTTTCCATCTCTTTGCGCC-3′, PyroSeq_MYB2_3, 5′-TGTTTTCCATCTCTTTGCGCC-3′. Pyrosequencing reaction was performed using PyroMark sequencer (Qiagen, Valencia, CA) in the Core Facility at The University of Texas at Austin. Small RNA blot analysis Total RNA (25 μg per sample in cotton and 10 μg per sample in Arabidopsis ) was prepared and electrophoresed in a 15% denaturing polyacrylamide gel containing 8 M of urea (National Diagnostics, Atlanta, GA). The RNA was transferred to Amersham Hybond-N+ nylon membranes (GE Healthcare, Piscataway, NJ, USA) and crosslinked with auto-UV. DNA oligonucleotide probes were: anti-ghmiR828, 5′-TCTTGCTCAAATGAGTATTCTACCTGT-3′; anti-sense-GhmiR858, 5′-TCAGGTCGAACAGACAATGAA-3′; MYB2-Tas 3′D8-Probe: 5′-GAATTCGTCCACATCAATGCT-3′; and U6, 5′-TGTATCGTTCCAATTTTATCGGATGT-3′. Each probe was labelled with γ 32P-ATP using T4 polynucleotide kinase (Promega, Madison, WI, USA). Prehybridization, hybridization and washing were performed following a published protocol [13] . After washing, the blot was exposed to a PhosphorImager screen (Fuji) for 3 h to overnight, and the screen was scanned using a Molecular Imager FX (Bio-Rad, Hercules, CA). The image was processed using the ImageQuant software (GE Healthcare, Piscataway, NJ). RNA ligase-mediated 5′ RACE RNA ligation-mediated rapid amplification of 5′ complementary DNA ends (5′ RACE) was conducted with GeneRacer kit (Invitrogen, Carlsbad, CA) to map the cleavage sites of target transcripts. Total RNA (4 μg) from cotton ovules (−3, 0, +3 DPA) and fibres (10 DPA) was ligated to a 5′ RACE RNA adapters without the treatment of calf intestine alkaline phosphatase. The first-strand cDNA was reverse transcribed using GeneRacer Oligo dT primer. A pool of non-gene-specific 5′ RACE products was generated using the GeneRacer 5′ primer (5′-CGACTGGAGCACGAGGACACTGA-3′) and the GeneRacer 3′ primer (5′-GCTGTCAACGATACGCTACGTAACG-3′). Gene-specific 5′ RACE amplifications were performed using the GeneRacer 5′ nested primer (5′-GGACACTGACATGGACTGAAGGAGTA-3′) and gene-specific primer (GhMYB2-NS-R: 5′-TACCATTGCTAATGGATCCTGTTGAT-3′). The 5′ RACE products were cloned, and 15–50 inserts were sequenced and analysed. Quantitative RT–PCR analysis Total RNA (1 μg) per sample was reverse transcribed to make cDNAs using the Omniscript RT Kit (Qiagen, Valencia, CA) and oligo dT primer. The qRT–PCR reaction was conducted in a 15 μl reaction containing 7.5 μl of FastStart Universal SYBR Green master (Rox) (Roche, Indianapolis, IN), 1 μM of forward and reverse primers in a 7500 Real-Time PCR system (Applied Biosystems, Carlsbad, CA). Amplification of cotton HISTONE H3 (AF024716; GhHIS3-F, 5′-GGCATACCTTGTGGGTCTTTTTGA-3′ and GhHIS3-R, 5′-CTACCACTACCATCATGGC-3′) and Arabidopsis UBQ10 (AT4G05320; UBQ10-F, 5′-CACACTCCACTTGGTCTTGCGT-3′ and UBQ10-R, 5′-TGGTCTTTCCGGTGAGAGTCTTCA-3′) were used to normalize the amount of gene-specific RT–PCR products. The MYB2 RT primer pair (MYB2-RTR, 5′-GGAGGAAGTTTGTTCTGTTCTGAC-3′ and MYB2-RTF: 5′-GCTGAGGAAGATAGATTGGC-3′) was used to amplify MYB2 transcripts. All reactions were performed in three technical replications using a dissociation curve to control the absence of primer dimers in the reactions. The amplification data were analysed using ABI7500 SDS software (version 1.2.2), and the relative expression levels (fold changes) were calculated using the standard control in each reaction. Ta-siRNA target prediction Ta-siRNA target prediction was performed on psRNATarget: A Plant Small RNA Target Analysis Server ( http://www.plantgrn.noble.org/psRNATarget/?dowhat=Citation ) [33] . Accession codes : Accession numbers of the MYB2 sequences deposited in the GenBank nucleotide database are JQ868555 ( G. arboreum L., A2); JQ868556 ( G. hirsutum L. TM-1_A); JQ868557 ( G. hirsutum L. TM-1, N1_A); JQ868558 ( G. thurberi , D1); JQ868559 ( G. raimondii , D5); JQ868560 ( G. hirsutum L. TM1_D); JQ868561 ( G. hirsutum L. TM-1, N1_D). How to cite this article : Guan, X. et al. miR828 and miR858 regulate homoeologous MYB2 gene functions in Arabidopsis trichome and cotton fibre development. Nat. Commun. 5:3050 doi: 10.1038/ncomms4050 (2014).